Ultrasonic hammer produces hot spots in solids Mechanical action can produce dramatic physical and mechanochemical effects when the energy is spatially or temporally concentrated. An important example of such phenomena in solids is the mechanical initiation of explosions, which has long been speculated to result from ‘hot spot’ generation at localized microstructures in the energetic material. Direct experimental evidence of such hot spots, however, is exceptionally limited; mechanisms for their generation are poorly understood and methods to control their locations remain elusive. Here we report the generation of intense, localized microscale hot spots in solid composites during mild ultrasonic irradiation, directly visualized by a thermal imaging microscope. These ultrasonic hot spots, with heating rates reaching ~22,000 K s −1 , nucleate exclusively at interfacial delamination sites in composite solids. Introducing specific delamination sites by surface modification of embedded components provides precise and reliable control of hot spot locations and permits microcontrol of the initiation of reactions in energetic materials including fuel/oxidizer explosives. The connection between the mechanical and the chemical worlds has both historical roots [1] and recent resurgence [2] , [3] , [4] , [5] . The concentration and conversion of diffuse mechanical energy at spatially confined regions of micrometre or even nanometre scale can result in intense localized heating (that is, formation of hot spots), especially in liquids and gels [6] , [7] , [8] , [9] , [10] . To study the spatial concentration of mechanical energy, one must have a means of energy localization at rates faster than thermal dissipation, control over its location and a ready method for time-resolved imaging of its formation and decay. Such investigations in solids (and especially in energetic materials, EMs), however, have proven to be difficult due to the complexity of material microstructures, chemical reactivity of the solids and short lifetimes of transient hot spots [10] , [11] . A classic example of mechanochemical processes in solid materials is the mechanical initiation of explosions (for example, by impact or shock), which has been intensively studied for more than a century [11] . The process has been widely presumed to involve hot spot formation within the EM by thermo-mechanical energy deposition at specific microstructures [11] , [12] , [13] , [14] , [15] . Direct experimental evidence for such hot spots, however, is so far exceptionally limited, the mechanisms for their formation are poorly understood and one’s ability to image and control hot spot locations remains elusive [16] , [17] . Typical solid explosives are composites of EM crystals with polymer binders [18] . Multiple mechanisms may lead to hot spot formation in these structures, such as shear banding of crystals, compression of voids, interfacial friction and triboelectric discharge [13] . Although model calculations have suggested that interstitial regions between crystals are critical locations for hot spot generation [18] , [19] , it is still difficult to identify specific contributions from multiple potential mechanisms. Furthermore, attempts to observe hot spots in solids are trapped in a dilemma: a mechanical impact strong enough to create intense energy concentration also crushes and destroys the microstructure of the material. The whole process occurs in microseconds, which is too fast to be captured by typical temporally and spatially resolved thermal imaging techniques (~100 frames per second) [20] . To improve our understanding of mechanochemical processes in solid structures, a new method that allows the imaging of thermomechanical energy deposition in solids is clearly needed. In this work, we have generated and imaged thermal–mechanical events in solids by applying ultrasonic irradiation as an alternative source of mechanical energy. With frequencies ranging from 20 kHz to 20 MHz, ultrasound can apply thousands to millions of small impacts repetitively into the material instead of a one-time powerful shock from conventional mechanical impact. The energy deposition process is therefore less destructive and also extends over a longer time period. As a delocalized mechanical energy, ultrasound induces acoustic cavitation in liquids and the resulting bubble collapse can generate micron-sized hot spots reaching temperatures and pressures of 15,000 K and 1,000 bar with an even hotter plasma core [8] , [21] , [22] , [23] . Ultrasound is also used for welding, a widely applied industrial technology; substantial frictional heating occurs at defined frictional contact points between two pieces of materials, although the process is highly empirical [24] , [25] . In contrast, ultrasound passing through bulk solid structures does not generally induce significant heating, with only very weak energy concentration at defects, with consequent heating limited to only a few K [26] , [27] . We show here that spontaneous and intense ultrasonic hot spots can be created inside solid materials, in particular polymer composites. The formation of such hot spots closely correlates with specific local structures in the composites and the modification of these structures leads to rational control of the microscale hot spots. This control, in turn, produces spatially and temporally definable thermal reactions in EMs, including fuel/oxidizer type explosives. Model composite systems and experimental design To avoid the complex interplay among various structural features (that is, mechanical discontinuities), we started with a simplified model that retains only the essential elements of a typical composite: a continuous polymer matrix, solid inclusions and, naturally, the interfaces between them. Particulates, either as a crystal or an amorphous particle, were sparsely embedded into the middle of a homogeneous polymer slab ( Fig. 1a,b and Supplementary Fig. 1a,b ). We could further control the interfacial mechanical and chemical properties of the material by surface modification of the embedded particulates. Ultrasound was delivered to the composite sample by pressing a vibrating ultrasonic horn against the slab surface, essentially an ultrasonic hammer (both the horn amplitude and the applied static pressure were adjustable; Supplementary Fig. 2 ), while a mid-wavelength infrared (MWIR) video microscope imaged thermal events inside the material (for thermographic calibration, see Methods and Supplementary Fig. 3 ). We have previously described the MWIR microscope for visualization of heating in solids during laser irradiation [28] , [29] . 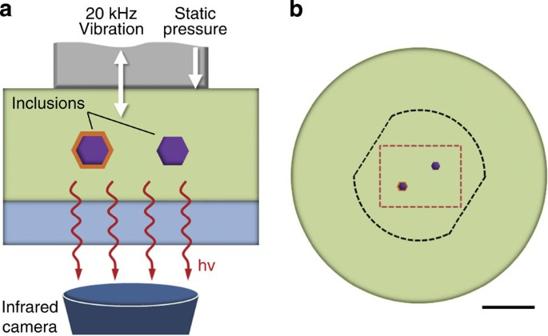Figure 1: Model composite system and experimental design. (a) Cross-sectional schematic showing a polymer slab (green) with a surface-modified inclusion and a pristine inclusion. An ultrasonic hammer is created by pressing a titanium rod vibrated at 20 kHz against the sample at a controlled pressure and the thermal emission from the sample is imaged through a sapphire window (blue). (b) Planar view of the same composite; area covered by the ultrasonic hammer, black dashed line; MWIR microscope image area, red dashed line. Scale bar, 5 mm. Figure 1: Model composite system and experimental design. ( a ) Cross-sectional schematic showing a polymer slab (green) with a surface-modified inclusion and a pristine inclusion. An ultrasonic hammer is created by pressing a titanium rod vibrated at 20 kHz against the sample at a controlled pressure and the thermal emission from the sample is imaged through a sapphire window (blue). ( b ) Planar view of the same composite; area covered by the ultrasonic hammer, black dashed line; MWIR microscope image area, red dashed line. Scale bar, 5 mm. Full size image Our technique for generating ultrasonic hot spots is extremely versatile and works well for a diverse range of composites. Polydimethylsiloxane (PDMS) was chosen as the polymer matrix for most of our studies because of its chemical inertness and thermal stability; we have also used cross-linked hydroxy-terminated polybutadiene (HTPB). Both polymers are common binders of EMs. We have examined several solid inclusions covering a wide variety of chemical reactivities and physical properties, including sucrose, NaCl, RDX (cyclotrimethylenetrinitramine), PBX (polymer-bonded explosives), ammonium nitrate and Teflon cubes. Effect of interfacial coating on hot spot generation As sucrose is a widely used simulant for EMs, our initial studies began with sucrose crystal inclusions embedded in PDMS. Under mild ultrasonic irradiation (that is, 44 μm peak-to-peak amplitude and 970 kPa static pressure), bulk heating of the polymer matrix is slow (~60 K s −1 ) and no localized heating occurs at the interfacial structures. To our surprise, however, if the sucrose crystals were coated with a thin liquid layer, for example, polyethylene glycol (PEG, molecular weight ~600 g mol −1 ), intense hot spots developed on these crystals under the same condition. As Fig. 2a,b shows, hot spot generated and reached more than 600 K in 60 ms on the PEG-coated sucrose inclusion. In sharp contrast, the polymer matrix and the pristine crystal embedded were barely heated during this period. The maximum heating rate of the hot spot reached 22,000 K s −1 ( Fig. 3 and Supplementary Fig. 4 ), on par with that of tissue ablation by typical surgical lasers. We estimate the energy conversion rate on the PEG-coated crystal surface to be 1.4 kW cm −2 , two orders higher than the bulk heating power of the polymer matrix, which is only ~13 W cm −2 at the horn surface (see Methods and Supplementary Fig. 5 for details of the calculations). The hot spot dynamics can be controlled by adjusting the ultrasound intensity. Under weaker ultrasonic irradiation (that is, 27 μm amplitude and 300 kPa static pressure), the development of hot spots took longer, nearly 200 ms ( Fig. 2c,d , Fig. 3 and Supplementary Movie 1 ). Similar hot spot dynamics were also consistently reproduced using a variety of other material compositions ( Supplementary Fig. 6 ), including ammonium nitrate, PBX and RDX ( Supplementary Fig. 7 ), showing that a liquid coating at the polymer–crystal interface serves as a nucleation site for intense localized hot spot generation. Changing the viscosity of the liquid coating from PEG (10.5 cSt) to glycerol (141.2 cSt), to non-cross-linked HTPB (1,500 cSt) does not lead to significant change in the hot spot dynamics ( Fig. 2c,d and Supplementary Fig. 6c–f ); thus, the properties of the thin liquid coating are not determinants of the hot spot characteristics. 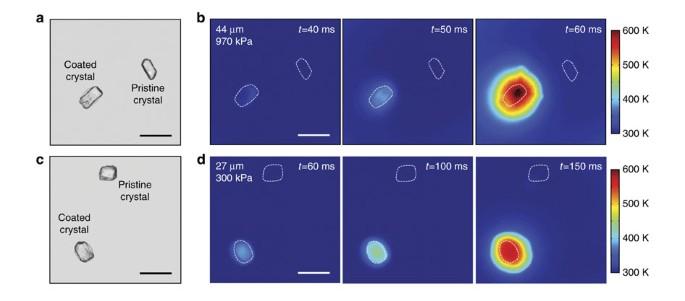Figure 2: Hot spot generation from surface-coated inclusions. (a) Optical micrograph of a composite of two sucrose crystals (one PEG-coated) embedded in PDMS and (b) thermographs of the sample inaduring ultrasonic irradiation (44 μm amplitude, 970 kPa applied pressure). Crystal locations are marked with dashed lines. (c) Optical micrograph of a second PDMS–sucrose composite with one of the sucrose crystal coated by PEG and (d) thermographs of the sample ineduring ultrasonic irradiation (27 μm amplitude, 300 kPa applied pressure). Scale bars, 1 mm (for all). Figure 2: Hot spot generation from surface-coated inclusions. ( a ) Optical micrograph of a composite of two sucrose crystals (one PEG-coated) embedded in PDMS and ( b ) thermographs of the sample in a during ultrasonic irradiation (44 μm amplitude, 970 kPa applied pressure). Crystal locations are marked with dashed lines. ( c ) Optical micrograph of a second PDMS–sucrose composite with one of the sucrose crystal coated by PEG and ( d ) thermographs of the sample in e during ultrasonic irradiation (27 μm amplitude, 300 kPa applied pressure). Scale bars, 1 mm (for all). 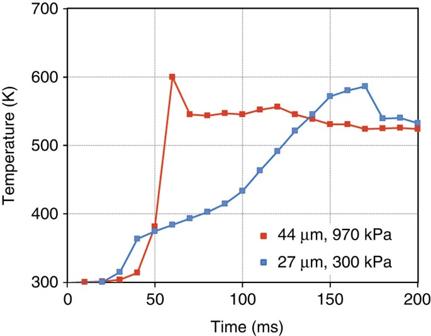Figure 3: Hot spot dynamics under different ultrasound intensities. Temperature evolution of the hot spots on the coated crystals inFig. 2a,c, respectively. Temperature was averaged from a 200 μm × 200 μm area at the centre of the hot spots for both samples. Full size image Figure 3: Hot spot dynamics under different ultrasound intensities. Temperature evolution of the hot spots on the coated crystals in Fig. 2a,c , respectively. Temperature was averaged from a 200 μm × 200 μm area at the centre of the hot spots for both samples. Full size image We can rule out several possible mechanisms that have been proposed for hot spot formation under mechanical stimuli. Cavitation in liquids or gels, for example, can induce gas-phase hot spots, but that does not apply to our composite solids: indeed, we do not observe heating from pure PEG liquid inclusions in a PDMS matrix ( Supplementary Fig. 8 ). We also cannot invoke particle breakage or shear banding of crystals as a mechanism for hot spot formation in these composites: if we stopped the sonication shortly after hot spots were initiated, no damage to the bulk crystals occurred ( Supplementary Fig. 9 ). In addition, as these are not EMs, a triboelectric discharge cannot account for our observed hot spot formation. Experimental evidence of interfacial delamination mechanism We believe that it is the interfacial delamination between the solid inclusion and the polymer that serves as nucleation sites for ultrasonic hot spots through frictional heating; local frictional heating has previously been speculated to occur under shockwave impact [13] , [19] , [30] , [31] . As shown in Fig. 4 , we examined the mechanical effects of sonication on solid composites with NaCl crystal inclusions that were coated either with liquid PEG or a solid film of polytetrafluoroethylene (PTFE, specifically Teflon-AF). During the development of an intense (~600 K) hot spot, a PEG-coated NaCl crystal sustained no substantial damage, but nevertheless showed a smoothing of its surface morphology ( Fig. 4a,b ), which suggests the existence of abrasive actions at the crystal–polymer interfaces. In contrast, we did not observe such morphological alteration on uncoated NaCl crystal inclusions after sonication. To exclude the possible interference from nonlinear acoustic effects in liquids (for example, cavitation and micro-streaming), we also made composites with NaCl crystal inclusions coated by a solid film (<2 μm thick, Supplementary Fig. 1c,d ) of PTFE. PTFE has low surface energy and therefore prevents adhesion between the inclusion and the polymer much as a liquid coating. Localized hot spots also evolve on the PTFE-coated crystal under ultrasonic irradiation, in quite similar dynamics and intensity to those generated on the PEG-coated NaCl crystals ( Fig. 4c,d ). Interestingly, we were also able to observe tearing and wrinkling of the PTFE coating after sonication, as direct evidence of interfacial friction ( Fig. 4e,f ). 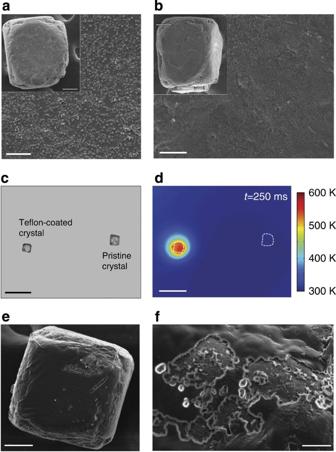Figure 4: Ultrasonic effects at the interface. (a) Scanning electron micrograph (SEM) of a pristine NaCl crystal (inset; scale bar, 100 μm) and a close-up of its surface (scale bar, 20 μm). (b) SEM of the same NaCl crystal (inset; scale bar, 100 μm) and its surface (scale bar, 20 μm) after formation of a 600-K hot spot, generated with PEG coating in a PDMS matrix, under the same condition as inFig. 2d. (c) Optical micrograph of a PDMS composite embedded with a PTFE-coated NaCl crystal and a pristine NaCl crystal (scale bar, 1 mm), and (d) thermograph of the sample when sonicated under the same conditions as inFig. 2d. (e) SEM of the PTFE-coated NaCl crystal after ultrasonic irradiation (scale bar, 100 μm) and (f) a close-up of the upper right quadrant ofeshowing the deterioration of the PTFE coating (scale bar, 20 μm). Figure 4: Ultrasonic effects at the interface. ( a ) Scanning electron micrograph (SEM) of a pristine NaCl crystal (inset; scale bar, 100 μm) and a close-up of its surface (scale bar, 20 μm). ( b ) SEM of the same NaCl crystal (inset; scale bar, 100 μm) and its surface (scale bar, 20 μm) after formation of a 600-K hot spot, generated with PEG coating in a PDMS matrix, under the same condition as in Fig. 2d . ( c ) Optical micrograph of a PDMS composite embedded with a PTFE-coated NaCl crystal and a pristine NaCl crystal (scale bar, 1 mm), and ( d ) thermograph of the sample when sonicated under the same conditions as in Fig. 2d . ( e ) SEM of the PTFE-coated NaCl crystal after ultrasonic irradiation (scale bar, 100 μm) and ( f ) a close-up of the upper right quadrant of e showing the deterioration of the PTFE coating (scale bar, 20 μm). Full size image Essentially, both a PTFE film and a liquid coating serve as nucleation sites for hot spots formation: they delaminate the particle–polymer interface, which allows relative motion between the two components on exposure to ultrasound. Once the inclusion and polymer are free to oscillate relative to one another, frictional heating dissipates the ultrasonic energy at the interface and generates hot spots. Compared with interfacial delamination, the bulk properties of the composite are much less important: hot spots are still observed when a NaCl crystal is replaced by a pure PTFE cube or when the PDMS matrix is replaced by HTPB ( Supplementary Fig. 6g–j ). Micro control of thermal reactions in EMs Hot spots, once initially formed in EMs, could cool down, cause slow burning or initiate detonation of the EM, depending on the hot spots’ sizes and temperatures. One might have imagined that hot spots could arise during ultrasonic irradiation at solid particle–particle interfaces or at voids, pores or cracks in the EM. However, we find that interfacial delamination is the dominant mechanism for ultrasonic hot spot formation and this permits us unprecedented control and confinement of thermal processes in a solid composite, especially EMs. By introducing localized surface modifications during material fabrication, we can preset precise locations for energy concentration and thereby control where explosions initiate in model solid EMs. We prepared PDMS composite samples with high loadings of RDX crystal, which inherently had large numbers of inter-crystal contacts; we put a liquid coating around specific RDX inclusions only. As shown by Fig. 5a , three RDX crystals were PEG-coated out of the ~100 crystals in the 0.25-cm 2 area of the PDMS composite. Under ultrasonic irradiation, hot spots arose simultaneously and exclusively at the three PEG-coated crystal sites. The hot spots then grew explosively, causing a thermal reaction to spread through the rest of the material ( Fig. 5b and Supplementary Movie 2 ). We can provide the same control over hot spot locations in samples with a real PBX (PBX-9407) that contained voids, pores and cracks; the presence of such complex microstructures did not compete with interfacial delamination for hot spot formation ( Supplementary Fig. 7e,f ). Recent work has examined ultrasonic heating of EMs (mostly with small temperature rises) and analysed its frequency dependence [32] , [33] . 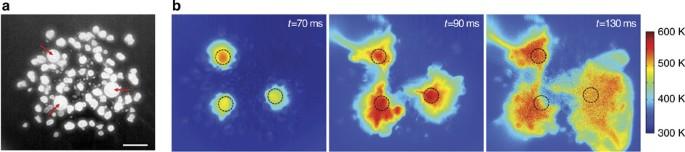Figure 5: Control of initiation locations in a composite explosive. (a) Infrared image showing ~100 RDX crystals embedded in a PDMS matrix, and the three crystals indicated by red arrows were coated with PEG. Scale bar, 1 mm. (b) Thermographs of the area inasonicated under the same conditions as inFig. 2bare displayed for 70, 90 and 130 ms. Original locations of the three coated crystals are outlined in black in all thermographs. Figure 5: Control of initiation locations in a composite explosive. ( a ) Infrared image showing ~100 RDX crystals embedded in a PDMS matrix, and the three crystals indicated by red arrows were coated with PEG. Scale bar, 1 mm. ( b ) Thermographs of the area in a sonicated under the same conditions as in Fig. 2b are displayed for 70, 90 and 130 ms. Original locations of the three coated crystals are outlined in black in all thermographs. Full size image The generation of ultrasonic hot spots can also be used to control the reactions of multiple components, for example, fuel/oxidizer explosives. We have applied ultrasound to trigger a vigorous inter-crystal reaction between sucrose and potassium chlorate, which are widely used for home-made explosives. As shown in Fig. 6a , the two solid particles surrounded by a layer of PEG were in close contact with each other in the PDMS matrix. Moderate ultrasonic irradiation generated localized heating of the two crystals through the same delamination mechanism, which then caused a runaway deflagration with the rapid release of hot gaseous products ( Fig. 6b–d ). The power of the inter-crystal reaction is evident from the size of the gas pocket created on the material ( Fig. 6b , t =80 ms, and Fig. 6c ). Noticeably, the reaction between the fuel and oxidizer can also occur when the two components are embedded in proximity to each other, but not in direct contact. A hot spot induced on either inclusion separately will grow and deflagration occurs when the hot spot expands to include the other inclusion. 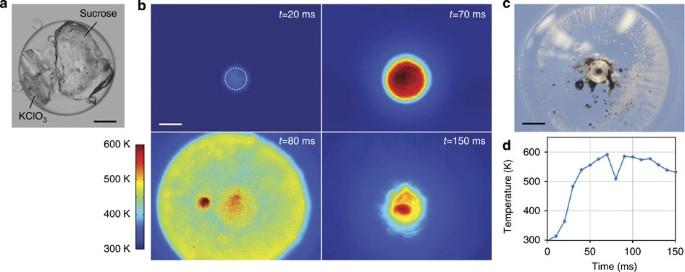Figure 6: Ultrasonic initiation of an inter-crystal fuel/oxidizer runaway reaction in a solid matrix. (a) Optical micrograph showing a PDMS composite with closely contacted PEG-coated sucrose and KClO3crystals as inclusions (scale bar, 200 μm). (b) Thermographs of the sample sonicated under the same conditions as inFig. 2d. The original location of the two embedded crystals is indicated by the dashed line in the thermal image at 20 ms. (c) Photograph of the same area after sonication showing a gas pocket. (d) Temperature evolution of the hot spot. Temperature was averaged from a 200 μm × 200 μm area at the centre of the hot spot. Figure 6: Ultrasonic initiation of an inter-crystal fuel/oxidizer runaway reaction in a solid matrix. ( a ) Optical micrograph showing a PDMS composite with closely contacted PEG-coated sucrose and KClO 3 crystals as inclusions (scale bar, 200 μm). ( b ) Thermographs of the sample sonicated under the same conditions as in Fig. 2d . The original location of the two embedded crystals is indicated by the dashed line in the thermal image at 20 ms. ( c ) Photograph of the same area after sonication showing a gas pocket. ( d ) Temperature evolution of the hot spot. Temperature was averaged from a 200 μm × 200 μm area at the centre of the hot spot. Full size image We have successfully demonstrated that ultrasound, as a mild source of mechanical energy, is able to generate intense hot spots in composite solids, and that we can control both the location and the dynamics of these hot spots. Sites of delamination between solid inclusions and the polymer matrix nucleate local frictional heating from relative motion of the polymer against the inclusion and initiate the formation of hot spots. The delamination can be a thin liquid coating, a surface treatment of the solid inclusion that prevents adhesion of the polymer, or a non-wettable solid (for example, a low surface energy material such as Teflon). The predominant contributor to the dynamics of hot spot formation is the ultrasonically induced motion of the matrix relative to the inclusion: roughly speaking, the hot spot dynamics are not substantially affected by the choice of solid inclusion or by the method of delamination. The hot spot is, however, strongly affected by the ultrasonic intensity. The ability to generate, image and manipulate hot spots in solids under ultrasonic irradiation provides a new platform to study mechanical energy concentration and to correlate such concentrations with local structural features. As a direct application, these ultrasonic hot spots are capable of initiating localized thermal reactions of EMs on the microscale. The fact that interfacial delamination dictates ultrasonic hot spot generation even in the presence of complex microstructures (that is, crystal contacts, voids, pores and cracks) provides a significant advantage over impact initiation of EMs: the dynamics of thermal initiation can be spatially controlled independently of composition or explosive microstructure. One might even speculate that control of local hot spot formation may provide methods to alter the overall rates of reactions in solids so that EMs may be driven into a slow decomposition rather than deflagration or detonation. Ultrasonic irradiation can also serve as a method to identify delamination defects in small samples from batch production of EM, permitting more reliable production of mechanically stable, impact-insensitive EM for critical applications. Although runaway exothermic reactions are easier to observe, ultrasonic hot spots should also be able to drive a much wider range of chemical processes in solids, regardless of the enthalpy of the reaction itself. The control of localized heating in solids is not only an issue for EM initiation, but also has general applicability to the transformation and fabrication of microstructured solids. Solid-state sonochemical reactions of potential future interest include redox reactions of metal ions, electrocyclic reactions of π -systems, self-healing materials (for example, in situ polymerizations) and mechanochemical depolymerizations. The last of these, indeed, has seen significant recent work ranging from depolymerization of vulcanized rubber [34] , [35] to cleavage of polymers at synthetically designed mechanophores embedded in the middle of the polymer chain [2] , [3] , [36] , [37] . General notes Sylgard 182 two-part PDMS kit was purchased from Dow Corning. Teflon AF solution (grade 601S1-100-6) was purchased from DuPont and the perfluoro solvent Fluorinert FC-770 was purchased from 3M. RDX crystals and PBX-9407 (Teledyne Technologies Inc.) were obtained from Dr Dan Hooks of Los Alamos National Laboratory. All other chemicals were purchased from Aldrich and used without further treatment unless otherwise noted. All crystals, except RDX and PBX-9407, were ground by a mortar and pestle, and were sifted with an ultrasonic sifter (ATM Corp.) to prepare solid particulates with diameters of 250–500 μm. RDX crystals of the same size range are hand picked with tweezers and PBX particles were cut from a pellet using a razor blade. Scanning electron micrographs were obtained on a JEOL 6060LV instrument operating at 10 kV and a working distance of 10 mm. Samples were mounted via carbon tape and sputter coated with ~10 nm of Au/Pd before imaging. Optical micrographs were obtained on a Zeiss Axioskop optical/fluorescence microscope with no polarizers inserted. Composite sample preparation To coat a crystal with liquid, the crystal was directly dipped into PEG (Mn ~600) or other kinds of liquid as specified. For the PTFE coating of crystals, 6 wt% Telfon AF solution was first diluted by FC-770 perfluoro solvent to make a 1.5 wt% Teflon AF solution. NaCl crystals were dipped into the solution, air-dried on a glass slide for a few minutes and then baked at 120 °C and 160 °C for 15 min each; the procedure was repeated a second time to achieve a homogeneous coating ( Supplementary Fig. 1c,d ). All samples were composed of a composite layer containing the solid inclusions, sandwiched on top and bottom by layers of pure polymer ( Supplementary Fig. 1a,b ). PDMS (Sylgard 182) was mechanically mixed by a 10:1 wt. ratio (base/accelerator) and degassed under vacuum. The mixture was spread on a sapphire window (diameter 25.4 mm, Thorlabs) to make a homogeneous layer ~300 μm thick and was cured at 100 °C for 15 min. After cooling to room temperature, the second layer of PDMS, ~600 μm thick, was spread and inclusions were immersed with the help of a thin needle. After subsequent curing and cooling, the third layer of PDMS, ~600 μm thick, was spread and cured at 100 °C for 60 min. HTPB ( M n ~1,200), when used as a polymer matrix, were mechanically mixed in a 83:17 wt ratio with isophorone diisocyanate and cured at 100 °C for 4 h for each layer of the slab. Ultrasonic irradiation and MWIR imaging As shown by Supplementary Fig. 2 , a 20-kHz ultrasonic horn (CV-33, Sonics and Materials Inc.) was pressed against the sample slab by four springs of adjustable length; the sample holder has a view-hole for the MWIR microscopic imaging. The static pressure imposed on the sample was calculated by measuring the stiffness and extension of the springs. Horn amplitude was measured using an optical microscope. The tip of the horn was cleaned before every experiment, to ensure uniform contact with the sample. Irradiation pulses were typically from 0.1 to 1 s in duration and were initiated while the MWIR microscope (IRE-640M, Sofradir-EC Inc., controlled by NI Vision Acquisition Software) was taking frames at 100 Hz and 100 μs integration time. The MWIR camera has 640 × 512 cooled HgCdTe pixels with a 15-μm pitch, with sensitivity in the 3.7–4.8 μm range. Temperature calibration and thermograph generation The infrared emission intensity was correlated with the temperature by an empirical calibration curve based on PDMS ( Supplementary Fig. 3a ). The data points on the calibration curve were obtained by averaging the infrared emission intensities from an ~1-mm PDMS cube both at room temperature (298 K) and after heating to elevated temperatures. The heater was made by a roll of heating tape and the temperature inside was measured by a thermocouple. Normalized intensity ( NI ) of the PDMS cube at a specific temperature was obtained by the following equation where I(T) is the IR intensity at temperature T: Due to the complexity of non-black body emission models, a smooth calibration curve was instead obtained by directly fitting the data points with an empirical allometric function: The temperature calibration data points cover the full dynamic range of the MWIR camera without extrapolation. NI higher than 180 (corresponding to temperatures greater than ~600 K) approaches the dynamic range limit of the camera and therefore provides the upper limit of our thermometry. Infrared images were converted into thermographs using the equation (2) in MATLAB. The crystal inclusions in the composite sample have slightly different emissivities than the PDMS matrix and the emissivity difference may also change with temperature. Therefore, the temperature calculated from the above calibration curve in principal could deviate from actual value for the inclusions. By direct observation of inclusions in a uniformly heated polymer, we are able to estimate the error to be <20 K based on the infrared emission homogeneity of the composite samples at measured temperatures up to ~400 K ( Supplementary Fig. 3b,c ). Power calculation on hot spots and on the bulk material The power output at a hot spot is equivalent to the ultrasonic energy converted to heat at the polymer-inclusion interface per unit time, assuming there is only neglible additional heating from exothermic chemical reactions that may also occur. The amount of energy converted at the interface can be calculated from the volume, temperature and heat capacity of the hot spot. Therefore: where V , d , C are the volume, density and heat capacity of the crystal and the polymer, respectively, A surface is the surface area of the crystal and ▵ t is the time for the corresponding temperature rise ▵ T . Specifically, for the experiment in Fig. 2a,b , we assume that ultrasonic energy converted on the sucrose crystal surface (simplied to a 400 μm × 400 μm × 700 μm rectangular box) heats up 200 K over 10 ms for a depth into the crystal and into the surrounding polymer matrix of ~200 μm (for a graphic representation of the simplified model see Supplementary Fig. 5 ); this depth of heating is taken experimentally from the second to third frames of Fig. 2b . Using the following values: d sucrose =1.59 g cm −3 , d PDMS =1.03 g cm −3 , C p,sucrose =1.24 J g −1 K −1 and C p,PDMS =1.46 J g −1 K −1 , and using the equation above, we obtained a power value of ~1.4 kW cm −2 at the crystal surface. The energy conversion rate on the bulk material was calculated by the following equation: where A horn tip is the area of the tip in contact with the sample and h is the sample thickness. ▵ T is the average temperature increase on the bulk sample. At the experimental condition of Fig. 2b , when no hot spot is present, the heating rate of bulk polymer is ~60 K s −1 . Using h =1.5 mm, d PDMS =1.03 g cm −3 , C p,PDMS =1.46 J g −1 K −1 , the bulk heating power was estimated to be 13 W cm −2 at the horn surface. How to cite this article: You, S. et al. Ultrasonic hammer produces hot spots in solids. Nat. Commun. 6:6581 doi: 10.1038/ncomms7581 (2015).